GABA depolarizes immature neurons and inhibits network activity in the neonatal neocortexin vivo A large body of evidence from in vitro studies suggests that GABA is depolarizing during early postnatal development. However, the mode of GABA action in the intact developing brain is unknown. Here we examine the in vivo effects of GABA in cells of the upper cortical plate using a combination of electrophysiological and Ca 2+ -imaging techniques. We report that at postnatal days (P) 3–4, GABA depolarizes the majority of immature neurons in the occipital cortex of anaesthetized mice. At the same time, GABA does not efficiently activate voltage-gated Ca 2+ channels and fails to induce action potential firing. Blocking GABA A receptors disinhibits spontaneous network activity, whereas allosteric activation of GABA A receptors has the opposite effect. In summary, our data provide evidence that in vivo GABA acts as a depolarizing neurotransmitter imposing an inhibitory control on network activity in the neonatal (P3–4) neocortex. γ-Aminobutyric acid (GABA) is the main inhibitory neurotransmitter in the adult brain in vivo [1] , [2] . It has long been recognized that GABA A receptor (GABA A R)-mediated inhibition involves both conductance-based (shunting) and voltage-based (hyperpolarization) mechanisms. During the last three decades, it became increasingly clear that the latter component is developmentally regulated [3] . Specifically, GABA was shown to depolarize immature neurons in various parts of the central nervous systems of diverse animal species [4] . The developmental depolarizing-to-hyperpolarizing GABA shift is thought to reflect a developmental decline in intracellular chloride concentration ([Cl – ] i ) due to a differential expression/efficacy of plasmalemmal chloride-accumulating (for example NKCC1 [5] , [6] , [7] ) versus chloride-extruding (for example KCC2 (ref. 8 ) co-transporters [9] , [10] . By facilitating the generation of action potentials, GABA was further found to promote the generation of patterned network activity [3] , [11] , [12] , [13] , [14] , [15] . These data led to the suggestion that GABA, whose synapses assemble before the ones for glutamate [16] , acts as one of the major excitatory neurotransmitters of the developing brain, underlying the activity-dependent growth and differentiation of neurons as well as the assembly of synaptic circuits [17] , [18] , [19] . Owing to an increase in membrane conductance, depolarizing GABAergic inputs may modulate neuronal output in a complex and bidirectional manner. Whether excitatory or inhibitory effects on neuronal firing dominate eventually depends on multiple parameters (including membrane potential, reversal potential of GABA A R-mediated currents, action potential threshold [20] , timing and location of inputs [21] , [22] , [23] as well as previous neuronal activity [24] , [25] ). Although criticism [26] , [27] , [28] concerning the concept of depolarizing GABA has been largely invalidated in recent years [29] , [30] , [31] , [32] , [33] , supportive evidence from the intact mammalian brain is still lacking. In favour of a depolarizing GABA action in non-mammalian species in vivo , iontophoretic application of GABA or glycine was found to evoke somatic Ca 2+ transients (CaTs) in spinal neurons of zebrafish larvae [34] . In addition, gramicidin-perforated patch recordings showed that GABA depolarizes zebrafish retinal ganglion cells at an early developmental stage [35] . At present, only limited information is available on the intact mammalian brain. In agreement with a role for NKCC1 in the generation of neonatal network activity, intraperitoneal injection of the NKCC1 antagonist bumetanide was reported to reversibly abolish hippocampal sharp waves in freely moving rat pups [36] . On the other hand, NKCC1 appears to be dispensable for spindle burst activity in the neonatal rodent somatosensory cortex [37] . Moreover, local blockade of GABA A Rs disinhibited the generation of spindle bursts [37] but not gamma oscillations [38] , while systemic administration of GABA A R antagonists was found to induce epileptic seizures in neonatal rats [39] . On the basis of these findings, potential conclusions on cellular GABAergic effects in vivo are limited. Here we directly address the question of whether GABA is depolarizing in vivo in the intact neocortex of living neonatal mice. We focussed on the upper cortical plate (CP) at postnatal days (P) 3–4, since previous investigations from several laboratories have convincingly shown that, in vitro , GABA acts as a predominantly depolarizing neurotransmitter on CP neurons at this age [4] , [30] , [31] . Combining electrophysiological and optical methods with multiple pharmacological manipulations, our results demonstrate that GABA depolarizes the majority of immature neurons in vivo but controls neocortical network activity mainly through inhibition. GABA depolarizes the majority of CP neurons at P3–4 in vivo To address the question whether GABA depolarizes immature cortical neurons in vivo , we first conducted two-photon-targeted patch-clamp recordings in spontaneously breathing, head-fixed mice at P3–4 under isoflurane anaesthesia. Of note, all cells included in the analysis were identified as neurons on the basis of their ability to generate action potentials (see Methods). Whole-cell voltage-clamp recordings were performed to verify that a 5-s-long pressure application of GABA from an epidurally positioned patch pipette (hereafter referred to as puff application) efficiently activated GABA A Rs in recorded neurons. Indeed, GABA application resulted in a pronounced and completely reversible reduction in membrane resistance from 749±104 to 46±10 MΩ (one-way repeated-measures analysis of variance (ANOVA), with Huynh–Feldt correction: P <0.001, n =9 neurons, η p 2 =0.84; control versus GABA: P <0.001, GABA versus washout: P <0.01, control versus washout: P >0.95, post hoc Bonferroni-corrected pairwise comparisons; Fig. 1a,b ). In a separate set of experiments, we then asked whether the same application protocol is suited to initiate action potential firing in CP cells. Using cell-attached recordings in loose-seal ( n =7) and tight-seal ( n =5; seal resistance >1 GΩ) voltage-clamp modes, none of the tested neurons displayed action currents in response to puff-applied GABA, whereas all cells showed robust burst firing in response to puff-applied glutamate ( Fig. 1c,d ). Accordingly, the following experiments were carried out in the absence of voltage-gated Na + channel antagonists. To non-invasively assess the polarity of GABA-induced membrane potential changes, we next used cell-attached current-clamp recordings [30] , [40] . Among 15 neurons recorded ( n =12 cells in the CP, n =3 cells in the marginal zone), puff-applied GABA induced monophasic membrane depolarization in 10 neurons ( Fig. 1e,f and Supplementary Fig. 1 ). Hyperpolarization in response to GABA was observed in two cells (one of which displayed a biphasic, initially hyperpolarizing, then depolarizing response; corresponding to cell 10 in Fig. 1f ), and inconsistent responses with a tendency towards depolarization were found in an additional three cells (cells 6, 11 and 12 in Fig. 1f ). The mean change in the measured potential amounted to +6.7±1.5 mV and differed significantly from zero ( n =15 cells, P <0.001, one-sample t -test on null hypothesis: mean=0). Additional experiments at P25–27 revealed that GABA A R activation in the presence of the membrane-permeable carbonic anhydrase inhibitor 6-ethoxy-2-benzothiazolesulfonamide (EZA; 150 μM) failed to induce membrane depolarization in the majority of layer 2/3 neurons in juvenile mice (P25–27: Δ V =+1.2±1.2 mV, n =10; P3–4: Δ V =+6.7±1.5 mV, n =15; P <0.05, two-sample t -test; Supplementary Fig. 2 ). On the basis of direct electrophysiological evidence, we hence conclude that GABA depolarizes the majority of immature CP neurons at P3–4. 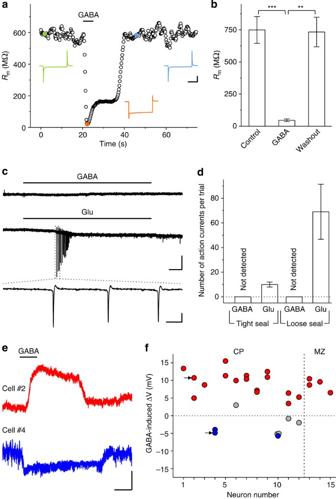Figure 1: GABAergic depolarization in immature neocortical neuronsin vivo. (a) Sample time course of membrane resistance (Rm,moving average over five trials) in response to GABA (100 mM, 5 s) puff-applied from an epidural pipette. Current responses to hyperpolarizing voltage steps (–10 mV) are shown as insets. Scale bars, 100 pA, 20 ms. (b) Quantification (n=9, cells one-way repeated-measures ANOVA, Huynh–Feldt-corrected:P<0.001;post hocBonferroni-corrected pairwise comparisons: control–GABA:P<0.001, GABA–washout:P<0.01, control–washout:P>0.95). (c) Cell-attached voltage-clamp recordings from a single neuron sequentially exposed to GABA (top; 100 mM, 5 s) and glutamate (Glu, bottom; 100 mM, 5 s). Scale bars, 20 pA, 500 ms (top) and 15 pA, 15 ms (bottom). (d) Number of action currents per trial in response to GABA and glutamate in tight-seal (n=5) and loose-seal (n=7) configurations. (e) Cell-attached current-clamp recordings obtained from two different neurons show that puff-applied GABA (100 mM, 5 s) evoked depolarization (cell #2) and hyperpolarization (cell #4), respectively. Scale bars, 5 mV, 5 s. (c,e) Electromagnetic artefacts due to valve opening/closure were clipped for clarity. (f) Quantification. Each cell was tested in one to three trials. Each symbol represents a single trial. Depolarizing responses are indicated by red symbols, hyperpolarizing responses by blue symbols. Grey-shaded symbols refer to trials with amplitudes lower than three times the s.d. of the baseline noise. Arrows point to trials shown ine. CP, cortical plate (n=12 cells); MZ, marginal zone (n=3 cells). (b,d) Data presented as mean±s.e.m. **P<0.01, ***P<0.001. Figure 1: GABAergic depolarization in immature neocortical neurons in vivo . ( a ) Sample time course of membrane resistance ( R m, moving average over five trials) in response to GABA (100 mM, 5 s) puff-applied from an epidural pipette. Current responses to hyperpolarizing voltage steps (–10 mV) are shown as insets. Scale bars, 100 pA, 20 ms. ( b ) Quantification ( n =9, cells one-way repeated-measures ANOVA, Huynh–Feldt-corrected: P <0.001; post hoc Bonferroni-corrected pairwise comparisons: control–GABA: P <0.001, GABA–washout: P <0.01, control–washout: P >0.95). ( c ) Cell-attached voltage-clamp recordings from a single neuron sequentially exposed to GABA (top; 100 mM, 5 s) and glutamate (Glu, bottom; 100 mM, 5 s). Scale bars, 20 pA, 500 ms (top) and 15 pA, 15 ms (bottom). ( d ) Number of action currents per trial in response to GABA and glutamate in tight-seal ( n =5) and loose-seal ( n =7) configurations. ( e ) Cell-attached current-clamp recordings obtained from two different neurons show that puff-applied GABA (100 mM, 5 s) evoked depolarization (cell #2) and hyperpolarization (cell #4), respectively. Scale bars, 5 mV, 5 s. ( c , e ) Electromagnetic artefacts due to valve opening/closure were clipped for clarity. ( f ) Quantification. Each cell was tested in one to three trials. Each symbol represents a single trial. Depolarizing responses are indicated by red symbols, hyperpolarizing responses by blue symbols. Grey-shaded symbols refer to trials with amplitudes lower than three times the s.d. of the baseline noise. Arrows point to trials shown in e . CP, cortical plate ( n =12 cells); MZ, marginal zone ( n =3 cells). ( b , d ) Data presented as mean±s.e.m. ** P <0.01, *** P <0.001. Full size image Lack of GABA-induced somatic CaTs at P3–4 Previous studies in neocortical brain slices have repeatedly demonstrated that activation of GABA A Rs can trigger a depolarization-dependent rise in intracellular free Ca 2+ concentration ([Ca 2+ ] i ) in immature neurons [5] , [13] , [30] , [41] . To investigate whether the same mechanism is functional in vivo , we next used two-photon Ca 2+ imaging in the upper CP ( Fig. 2a,b ). In an initial set of experiments, mice were administered the analgesic-sedative nitrous oxide to circumvent (I) potential complications of conventional anaesthetics (which are known to interfere with the generation of large-scale Ca 2+ waves in rodent pups [42] , [43] ) or (II) recordings in unanaesthetized mice [44] . In agreement with the observed lack of GABA-induced action potential firing (see above), we found that puff application of GABA (100 mM, for definition of the application time see Methods) from an epidurally positioned pipette mostly failed to evoke distinct somatic CaTs in glutamate-responsive cells ( Fig. 2c ). At P3–4, the GABA-induced relative change in fluorescence (Δ F / F 0 ) amounted to 0.01±0.00 ( P >0.15, n =204 cells from five mice, one-sample Wilcoxon-signed rank test on null hypothesis: median=0; Fig. 2d ). On the basis of a Δ F / F 0 threshold criterion (see Methods), one out of 204 cells was classified as responsive to GABA. Similar results were obtained when the duration of the GABA puff was prolonged by a factor of five (six out of 204 cells were classified as responsive to GABA; Δ F / F 0 =0.01±0.01, P >0.95, n =204 cells, one-sample Wilcoxon-signed rank test). Subsequent to the in vivo experiments, acute brain slices comprising the stained region were prepared and the experiment was repeated in vitro ( Supplementary Fig. 3a–f ). To reduce differences in effective concentrations of GABA and glutamate reaching the cells of interest, pipette concentrations of agonists were reduced (1 mM) and application times were adjusted such that amplitudes of glutamate-induced CaTs in vitro matched those in vivo (Δ F / F 0 in vivo : 1.45±0.03, n =204 cells, Δ F / F 0 in vitro : 1.46±0.02, n =407 cells from 10 slices and five mice, P >0.45, Mann–Whitney U -test; Supplementary Fig. 3e,f ). In line with data from naive slices [13] , [30] , puff-applied GABA triggered significant CaTs in glutamate-responsive cells (GABA-induced Δ F / F 0 : 0.40±0.01, P <0.001, n =407 cells from 10 slices and five mice, one-sample Wilcoxon-signed rank test on null hypothesis: median=0; Supplementary Fig. 3c–f ). When normalized to glutamate response amplitudes, GABA-induced Δ F / F 0 values differed significantly between cells within intact cortex and slice, respectively ( in vivo : 0.00±0.00, n =204 cells, in vitro : 0.29±0.01, n =407 cells, P <0.001, Mann–Whitney U -test). We next examined the effects of lower GABA concentrations (1 and 10 mM) and/or shorter application times (10% of t short ; see Methods) under isoflurane anaesthesia. However, GABA-induced somatic CaTs were not detected under these conditions (10 mM and t short : Δ F/F 0 =0.00±0.01; 10 mM and 10% of t short : Δ F/F 0 =0.00±0.00; 1 mM and t short : Δ F/F 0 =–0.02±0.01; 1 mM and 10% of t short : Δ F/F 0 =–0.01±0.00; none out of 44 cells from two mice was classified as responsive to GABA). Collectively, our data suggest that in vivo GABA does not efficiently activate voltage-gated Ca 2+ channels (VGCCs) at P3–4. 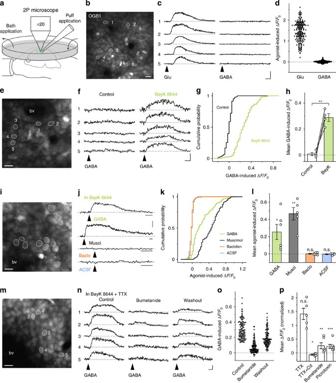Figure 2: GABA-induced somatic Ca2+transients in the presence of BayK 8644in vivo. (a) Experimental arrangement. (b,e,i,m) Two-photon fluorescence images of OGB1-stained CP cellsin vivo. Scale bars, 10 μm; bv, blood vessel. (c) Single-cell Ca2+responses to puff-applied glutamate (Glu; 100 mM, 0.3 s) and GABA (100 mM, 0.3 s). Scale bars, 1.5 ΔF/F0, 2.5 s. (d) ΔF/F0amplitude distributions. Each symbol represents a single cell (n=204 cells, five mice). (f) GABA-induced Ca2+responses in the absence (Control) and presence of BayK 8644 (20 μM). Scale bars, 0.5 ΔF/F0, 5 s. (g) ΔF/F0amplitude distributions (n=126 cells, four mice). (h) The mean ΔF/F0amplitudes per animal (P<0.01,n=4 mice, pairedt-test). (j) Ca2+responses (averages from 12 cells shown ini) to GABA (100 mM), Muscimol (Musci, 5 mM), Baclofen (Baclo, 5 mM) and ACSF. Note differences in time-axis scaling. Scale bars, 0.25 ΔF/F0, 5 s. (k) ΔF/F0amplitude distributions (GABA:n=172 cells; Muscimol:n=139 cells; Baclofen:n=172 cells; ACSF:n=139 cells). (l) The mean ΔF/F0amplitudes per animal (GABA:P<0.05,n=6 mice; Muscimol:P<0.01,n=5 mice; Baclofen:P>0.95,n=6 mice; ACSF:P>0.4,n=5 mice; one-sample Wilcoxon-signed rank tests). (n) GABA-induced Ca2+responses were sensitive to bumetanide (50 μM). Scale bars, 0.25 ΔF/F0, 5 s. (o) Single-cell GABA-induced ΔF/F0amplitude distributions (n=122 cells, six mice). (p) The mean GABA-induced ΔF/F0amplitudes per animal (normalized to control). GABA-induced Ca2+transients did not require voltage-gated Na+channels (TTX:P>0.15,n=5 mice) but were sensitive to antagonists of voltage-gated Ca2+channels (TTX+CdCl2:P<0.05,n=4 mice, Bonferroni-corrected pairedt-tests), NKCC1 (Bumetanide:n=6; repeated-measures ANOVA:P<0.001, Bonferroni test:P<0.01) and GABAAreceptors (Picrotoxin:P<0.001,n=7; pairedt-test). Picrotoxin and bumetanide were tested in the presence of TTX. (i–p) Experiments were performed in the presence of BayK 8644. (h,l,p) Data presented as mean±s.e.m. *P<0.05, **P<0.01, ***P<0.001, n.s., not significant. Figure 2: GABA-induced somatic Ca 2+ transients in the presence of BayK 8644 in vivo. ( a ) Experimental arrangement. ( b , e , i , m ) Two-photon fluorescence images of OGB1-stained CP cells in vivo . Scale bars, 10 μm; bv, blood vessel. ( c ) Single-cell Ca 2+ responses to puff-applied glutamate (Glu; 100 mM, 0.3 s) and GABA (100 mM, 0.3 s). Scale bars, 1.5 Δ F / F 0 , 2.5 s. ( d ) Δ F / F 0 amplitude distributions. Each symbol represents a single cell ( n =204 cells, five mice). ( f ) GABA-induced Ca 2+ responses in the absence (Control) and presence of BayK 8644 (20 μM). Scale bars, 0.5 Δ F / F 0 , 5 s. ( g ) Δ F / F 0 amplitude distributions ( n =126 cells, four mice). ( h ) The mean Δ F / F 0 amplitudes per animal ( P <0.01, n =4 mice, paired t -test). ( j ) Ca 2+ responses (averages from 12 cells shown in i ) to GABA (100 mM), Muscimol (Musci, 5 mM), Baclofen (Baclo, 5 mM) and ACSF. Note differences in time-axis scaling. Scale bars, 0.25 Δ F / F 0 , 5 s. ( k ) Δ F / F 0 amplitude distributions (GABA: n =172 cells; Muscimol: n =139 cells; Baclofen: n =172 cells; ACSF: n =139 cells). ( l ) The mean Δ F / F 0 amplitudes per animal (GABA: P <0.05, n =6 mice; Muscimol: P <0.01, n =5 mice; Baclofen: P >0.95, n =6 mice; ACSF: P >0.4, n =5 mice; one-sample Wilcoxon-signed rank tests). ( n ) GABA-induced Ca 2+ responses were sensitive to bumetanide (50 μM). Scale bars, 0.25 Δ F / F 0 , 5 s. ( o ) Single-cell GABA-induced Δ F / F 0 amplitude distributions ( n =122 cells, six mice). ( p ) The mean GABA-induced Δ F / F 0 amplitudes per animal (normalized to control). GABA-induced Ca 2+ transients did not require voltage-gated Na + channels (TTX: P >0.15, n =5 mice) but were sensitive to antagonists of voltage-gated Ca 2+ channels (TTX+CdCl 2 : P <0.05, n =4 mice, Bonferroni-corrected paired t -tests), NKCC1 (Bumetanide: n =6; repeated-measures ANOVA: P <0.001, Bonferroni test: P <0.01) and GABA A receptors (Picrotoxin: P <0.001, n =7; paired t -test). Picrotoxin and bumetanide were tested in the presence of TTX. ( i–p ) Experiments were performed in the presence of BayK 8644. ( h , l , p ) Data presented as mean±s.e.m. * P <0.05, ** P <0.01, *** P <0.001, n.s., not significant. Full size image For comparison, additional experiments were performed at P1 ( n =3 mice). Using the standard puff application duration ( t short ), 11 out of 117 cells (9.4%) were found to be responsive to GABA (versus 1 out of 204 cells (0.5%) at P3–4: P <0.001, Pearson’s χ 2 -test) and GABA-induced Δ F/F 0 amplitudes differed significantly from zero (Δ F / F 0 =0.07±0.01, P <0.001, one-sample Wilcoxon-signed rank test; Supplementary Fig. 4 ). Similar results were obtained when the duration of the GABA puff was prolonged by a factor of five (Δ F / F 0 =0.06±0.01, P <0.001, one-sample Wilcoxon-signed rank test; 11 out of 117 cells were classified as responsive to GABA at P1 versus 6 out of 204 cells at P3–4: P =0.013, Pearson’s χ 2 -test; Supplementary Fig. 4 ). These data show that (I) a significantly larger fraction of cells is responsive to GABA at P1 as compared with P3–4 and, at the same time, (II) the vast majority of cells (>90%) are non-responsive to GABA in both age groups. GABA-evoked CaTs in presence of BayK 8644 at P3–4 Previous investigations in acute brain slices revealed that GABA-mediated CaTs in CP cells mainly involve L-type VGCCs [5] whose activation threshold is considerably more positive than typical resting membrane potentials. Consequently, even moderate depolarizations might not affect [Ca 2+ ] i . We therefore aimed at increasing the detection sensitivity for depolarization by enhancing the VGCC-mediated Ca 2+ flux. To this end, we used BayK 8644, a well-characterized positive modulator of L-type VGCCs known to increase their mean open time and to shift the voltage dependence of activation towards more negative potentials [45] . In naive neocortical slices at P3–4, and in line with data from the olfactory bulb [46] , we found that BayK 8644 (20 μM) consistently increased the amplitude of GABA-induced CaTs in the upper CP (Δ F / F 0 in control: 0.35±0.09, Δ F / F 0 in BayK 8644: 0.79±0.07, P <0.01, n =5 slices, paired t -test; Supplementary Fig. 3g–j ). We next analysed the effect of BayK 8644 (20 μM) in vivo by superfusion of the exposed dura mater (hereafter referred to as bath application). We found that bath-applied BayK 8644 unmasked GABA-induced CaTs in vivo . The mean GABA-induced Δ F / F 0 values in glutamate-responsive cells were 0.01±0.01 in control and 0.29±0.03 in the presence of BayK 8644 ( P <0.01, n =4 mice with 126 cells, paired t -test; Fig. 2e–h ). We next examined whether CaTs induced by epidural puff application of GABA in the presence of BayK 8644 were sensitive to the conventional anaesthetic isoflurane. On average, amplitudes of GABA-mediated CaTs were not significantly affected (N 2 O: 0.28±0.04, isoflurane plus N 2 O: 0.24±0.17, P >0.8, n =3 mice with 92 cells, paired t -test). Since the addition of isoflurane increased mechanical recording stability, we used the latter anaesthetic regime for further pharmacological characterizations. In glutamate-responsive cells and in the presence of BayK 8644, GABA-mediated CaTs (Δ F / F 0 : 0.25±0.09, P <0.001, n =6 mice with 172 cells) were mimicked by the specific GABA A R agonist muscimol (5 mM; Δ F / F 0 : 0.47±0.07, P <0.001, n =5 mice with 139 cells, one-sample Wilcoxon-signed rank tests on null hypothesis: median=0; Fig. 2i–l ). In these experiments, the fraction of agonist-responsive cells (defined as Δ F / F 0 larger than three times the s.d. of single-cell amplitudes in response to puff-applied artificial cerebrospinal fluid (ACSF), that is, Δ F / F 0 >0.13) was 55% for GABA and 95% for muscimol. As expected, GABA- and muscimol-induced Δ F / F 0 values displayed a significant positive correlation (Spearman’s ρ =0.67, P <0.001, n =90 cells, only GABA-responsive cells included; Supplementary Fig. 5 ). In contrast, CaTs were not observed in response to the specific GABA B receptor agonist baclofen (5 mM; Δ F / F 0 : 0.00±0.01, P >0.95, n =6 mice with 172 cells) or ACSF alone (Δ F / F 0 : –0.00±0.00, P >0.4, n =5 mice with 139 cells, one-sample Wilcoxon-signed rank tests on null hypothesis: median=0; Fig. 2j–l ). Furthermore, in GABA-responsive cells, GABA-mediated CaTs were not reduced in amplitude by the voltage-gated Na + channel blocker tetrodotoxin (TTX, 3 μM; Δ F / F 0 : 142±21% of control, P >0.15, n =5 mice with 102 cells; Fig. 2p ), suggesting that action potential-dependent network excitation did not contribute to their generation. By contrast, GABA-mediated CaTs were completely abolished by the subsequent addition of the broad-spectrum VGCC antagonist CdCl 2 (200–300 μM), indicating the dependence on depolarization (Δ F / F 0 : –5.9±2.6% of control, n =4 mice with 82 cells, P <0.05, paired t -tests with Bonferroni correction; Fig. 2p ). In neocortical neurons in vitro , the Na + /K + /2Cl – co-transporter NKCC1 was previously shown to maintain [Cl – ] i above passive distribution [5] , [12] , [18] . In agreement with this, we found that bath application of the NKCC1 inhibitor bumetanide (50 μM) reduced the amplitudes of GABA-mediated CaTs in GABA-responsive cells to 26±11% that partially recovered to 67±9.0% during washout (one-way repeated-measures ANOVA: P <0.001, n =6 mice with 122 cells, η p 2 =0.86; control versus bumetanide: P <0.01; bumetanide versus washout: P <0.01, post hoc Bonferroni-corrected pairwise comparisons; Fig. 2m–p ). The latter experiments were conducted in the presence of TTX to inhibit recurrent excitation. Involvement of GABA A Rs was further corroborated by the observation that bath-applied GABA A R antagonist picrotoxin (250 μM) strongly reduced the amplitudes of GABA-evoked CaTs to 24±6.8% ( P <0.001, n =7 mice with 111 cells, paired t -test; four of seven mice were previously exposed to bumetanide; Fig. 2p ). Collectively, these data provide evidence for a depolarizing effect of GABA A R activation in the majority of CP cells in vivo at P3–4. Synaptic excitation depends on glutamatergic input We next sought to determine whether GABAergic synaptic activity is able to trigger action potential discharge in immature cortical cells. To address this question, we applied repetitive electrical stimulation (25 pulses, 50 Hz) via a low-resistance glass electrode positioned in the upper CP. First, we used two-photon Ca 2+ imaging ( Fig. 3a,b ) as a secondary readout of action potential firing [47] . With both GABAergic and glutamatergic transmission intact, electrical stimulation induced somatic CaTs in the vast majority of cells examined (70 out of 73 cells from three mice; 45 of these cells responded during each of three trials; Fig. 3c ). Bath application of ionotropic glutamate receptor antagonists (50 μM 6,7-dinitroquinoxaline-2,3(1H,4H)-dione (DNQX) plus 250 μM DL-2-amino-5-phosphonopentanoic acid (APV)) blocked stimulation-induced CaTs in all cells except one (cell #49; Fig. 3c ). The latter was probably activated in an antidromic manner since responses persisted even in the additional presence of the GABA A R antagonist gabazine (40 μM). These data suggest that GABAergic afferent stimulation alone is insufficient to induce somatic CaTs in upper CP cells. In line with this conclusion, local puff application of GABA from a pipette positioned within the CP also failed to induce somatic CaTs in upper CP cells ( Supplementary Fig. 6 ). 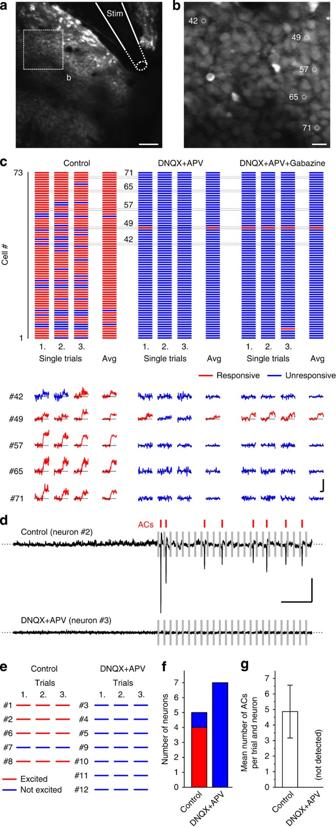Figure 3: Lack of somatic Ca2+transients and action potential discharge in response to GABAergic afferent stimulationin vivo. (a) Two-photon fluorescence image of OGB1-stained CP cellsin vivoafter positioning of an extracellular stimulation electrode (stim). Scale bar, 50 μm. (b) Field of view during recording as indicated by a dashed rectangle ina. Scale bar, 10 μm. (c) Top: for both single trials and averaged traces cells were independently classified as responsive (red) or unresponsive (blue) based on an amplitude-threshold criterion. Each stimulation trial consisted of 25 pulses delivered at 50 Hz. All cells included were tested in standard ACSF (Control, left), in the presence of DNQX (50 μM) plus APV (250 μM, middle) as well as in the presence of DNQX plus APV plus Gabazine (40 μM, right). Bottom: sample traces from five cells indicated inb. Note that DNQX plus APV blocked responses in all cells except one (#49). Scale bars, 0.5 ΔF/F0, 1 s. (d) Cell-attached voltage-clamp recordings from two different neurons in standard ACSF (Control) and in the presence of DNQX plus APV, respectively. Each repetitive electrical stimulation trial consisted of 25 pulses delivered at 50 Hz. Stimulation artefacts were blanked for clarity (grey bars). Action currents (ACs) are indicated by red vertical lines. Scale bars, 25 pA, 100 ms. (e) Summary plot of excited (red) and non-excited (blue) neurons (n=5 cells in control,n=7 cells in DNQX plus APV). (f) Absolute number of excited and non-excited neurons. (g) The mean number of action currents per neuron and trial. Data presented as mean±s.e.m. Figure 3: Lack of somatic Ca 2+ transients and action potential discharge in response to GABAergic afferent stimulation in vivo . ( a ) Two-photon fluorescence image of OGB1-stained CP cells in vivo after positioning of an extracellular stimulation electrode (stim). Scale bar, 50 μm. ( b ) Field of view during recording as indicated by a dashed rectangle in a . Scale bar, 10 μm. ( c ) Top: for both single trials and averaged traces cells were independently classified as responsive (red) or unresponsive (blue) based on an amplitude-threshold criterion. Each stimulation trial consisted of 25 pulses delivered at 50 Hz. All cells included were tested in standard ACSF (Control, left), in the presence of DNQX (50 μM) plus APV (250 μM, middle) as well as in the presence of DNQX plus APV plus Gabazine (40 μM, right). Bottom: sample traces from five cells indicated in b . Note that DNQX plus APV blocked responses in all cells except one (#49). Scale bars, 0.5 Δ F / F 0 , 1 s. ( d ) Cell-attached voltage-clamp recordings from two different neurons in standard ACSF (Control) and in the presence of DNQX plus APV, respectively. Each repetitive electrical stimulation trial consisted of 25 pulses delivered at 50 Hz. Stimulation artefacts were blanked for clarity (grey bars). Action currents (ACs) are indicated by red vertical lines. Scale bars, 25 pA, 100 ms. ( e ) Summary plot of excited (red) and non-excited (blue) neurons ( n =5 cells in control, n =7 cells in DNQX plus APV). ( f ) Absolute number of excited and non-excited neurons. ( g ) The mean number of action currents per neuron and trial. Data presented as mean±s.e.m. Full size image Single action potentials might escape detection in OGB1-based Ca 2+ imaging experiments [47] . We therefore performed additional two-photon-guided cell-attached recordings in the upper CP. All cells included in the analysis were identified as neurons on the basis of their ability to generate action potentials. With both GABAergic and glutamatergic transmission intact, repetitive electrical stimulation (25 pulses, 50 Hz) triggered action potential firing in four out of five neurons ( Fig. 3d–f ). The average number of action currents per trial and cell amounted to 4.9±1.7 ( n =5 neurons; Fig. 3g ). In contrast, in the presence of DNQX plus APV, electrical stimulation failed to initiate action potential firing in all neurons examined ( n =7 neurons; Fig. 3d–g ). In summary, we conclude that synaptically driven action potential firing at P3–4 in vivo is largely dependent on glutamatergic, but not GABAergic, input. Spontaneous neocortical network activity in vivo We next aimed at elucidating how GABA contributes to the generation of cortical network activity. To this end, we performed wide-field epifluorescence Ca 2+ imaging in mice (P3–4) expressing the genetically encoded Ca 2+ indicator GCaMP3 in cortical glutamatergic cells ( Emx1 IREScre :GCaMP3 LSL mice) [43] , [48] , [49] ( Fig. 4a,b ). For analysis, the field of view ( ∼ 1 mm 2 ) was subdivided into a regular grid of regions of interest (ROI; Fig. 4c ). When mice were anaesthetized with N 2 O, spontaneous network activity occurred in the form of spatiotemporal clusters of CaTs in all animals examined ( n =21 mice; Fig. 4b–d and Supplementary Movie 1 ). Single-cell two-photon Ca 2+ imaging in Emx1 IREScre :GCaMP3 LSL mice confirmed that Ca 2+ cluster activity also involves the upper CP ( n =5 mice; Supplementary Fig. 7a–d ). To correlate these Ca 2+ cluster events to previously reported electrophysiologically defined activity patterns, wide-band extracellular recordings (0.1–6,000 Hz) and wide-field Ca 2+ imaging were performed simultaneously ( n =4 mice). To this end, a low-resistance glass electrode was positioned in the upper CP under two-photon guidance ( Fig. 4e,f ). We found that Ca 2+ clusters occurring in proximity of the tip of the pipette were paralleled by distinct field potential changes ( Fig. 4g ). Wavelet-based time-frequency and fast Fourier transform (FFT) analysis revealed that, in the majority of cases, the latter consisted of spindle-shaped oscillations with a dominant frequency in the theta (4–8 Hz; occasionally and to a lesser extent alpha (8–13 Hz)) band, typically nested in a delta wave ( Fig. 4h ). Spindle-like oscillations were usually accompanied by rhythmic multiunit discharges that were phase-locked to the troughs of the spindle oscillation ( Fig. 4h ). In some cases, spindle-like oscillations were less obvious (<3 cycles) or not detectable and the delta component was dominant. Interestingly, in several cases, theta oscillations were simultaneously evident in the GCaMP3 signal (see events #1 and #2 in Fig. 4h ). In summary, the electrophysiological characteristics of Ca 2+ clusters agree well with those of previously reported spindle bursts in the visual cortex of neonatal rats [50] , [51] , [52] . 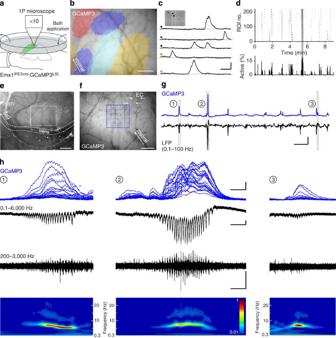Figure 4: Ca2+cluster activity in the neonatal occipital neocortexin vivo. (a) Experimental arrangement. (b) GCaMP3 fluorescence overlaid with area plots of four spatially confined cluster events (colour-coded). Binary area plots were calculated from ΔF/F0sequences (averaged over 10 frames) as maximum intensity projections thresholded at 25% of the peak amplitude. Scale bar, 200 μm. (c) Sample traces (ΔF/F0) from individual ROIs. Colour code refers to clusters inb. Inset corresponds to field of view as shown inb, and indicates positions of ROIs from which sample traces were obtained. Note the presence of several spatiotemporally distinct Ca2+clusters. Scale bars, 0.25 ΔF/F0, 2 s. (d) Top: Raster plot indicating times of peak of Ca2+transients from all individual ROIs. The time period shown incis highlighted in grey. Bottom: time-aligned plot of the fraction of active ROIs, obtained by summing peaks over moving windows 10 frames in length. (e)In vivoview of a craniotomy (∼1.2 mm2) over the occipital cortex. The field of view during recording (shown inf) is indicated by a dotted rectangle (trans, transverse sinus; sag, superior sagittal sinus; ch, margin of recording chamber). Scale bar, 500 μm. (f) GCaMP3 fluorescence image after positioning of an extracellular electrode (EC). Scale bar, 200 μm. (g) Time-aligned sample traces of GCaMP3 fluorescence (average of 25 ROIs shown infhigh-pass filtered at 0.01 Hz) and local field potential (LFP, band-pass-filtered at 0.1–100 Hz). Scale bars, 0.2 ΔF/F0, 200 μV, 50 s. LED synchronization pulses were clipped for clarity. (h) Time-aligned GCaMP3 fluorescence (top, overlaid for 25 ROIs shown inf), wide-band extracellular signal (0.1–6,000 Hz), multiunit activity (200–3,000 Hz) and Morlet wavelet spectrum for the three time intervals indicated ing. Scale bars, 0.2 ΔF/F0, 100 μV, 1 s. The asterisk in event 1 indicates a single blanked LED synchronization pulse. Figure 4: Ca 2+ cluster activity in the neonatal occipital neocortex in vivo . ( a ) Experimental arrangement. ( b ) GCaMP3 fluorescence overlaid with area plots of four spatially confined cluster events (colour-coded). Binary area plots were calculated from Δ F / F 0 sequences (averaged over 10 frames) as maximum intensity projections thresholded at 25% of the peak amplitude. Scale bar, 200 μm. ( c ) Sample traces (Δ F / F 0 ) from individual ROIs. Colour code refers to clusters in b . Inset corresponds to field of view as shown in b , and indicates positions of ROIs from which sample traces were obtained. Note the presence of several spatiotemporally distinct Ca 2+ clusters. Scale bars, 0.25 Δ F / F 0 , 2 s. ( d ) Top: Raster plot indicating times of peak of Ca 2+ transients from all individual ROIs. The time period shown in c is highlighted in grey. Bottom: time-aligned plot of the fraction of active ROIs, obtained by summing peaks over moving windows 10 frames in length. ( e ) In vivo view of a craniotomy ( ∼ 1.2 mm 2 ) over the occipital cortex. The field of view during recording (shown in f ) is indicated by a dotted rectangle (trans, transverse sinus; sag, superior sagittal sinus; ch, margin of recording chamber). Scale bar, 500 μm. ( f ) GCaMP3 fluorescence image after positioning of an extracellular electrode (EC). Scale bar, 200 μm. ( g ) Time-aligned sample traces of GCaMP3 fluorescence (average of 25 ROIs shown in f high-pass filtered at 0.01 Hz) and local field potential (LFP, band-pass-filtered at 0.1–100 Hz). Scale bars, 0.2 Δ F / F 0 , 200 μV, 50 s. LED synchronization pulses were clipped for clarity. ( h ) Time-aligned GCaMP3 fluorescence (top, overlaid for 25 ROIs shown in f ), wide-band extracellular signal (0.1–6,000 Hz), multiunit activity (200–3,000 Hz) and Morlet wavelet spectrum for the three time intervals indicated in g . Scale bars, 0.2 Δ F / F 0 , 100 μV, 1 s. The asterisk in event 1 indicates a single blanked LED synchronization pulse. Full size image Although the aforementioned measurements were acquired through the intact dura after surgical removal of the overlying bone, virtually identical Ca 2+ cluster activity was observed through the intact skull ( n =3 mice; Supplementary Fig. 7e–k ). In addition, similar spatiotemporal clusters of CaTs (although with moderately higher frequency and lower cluster size) were also apparent in the absence of N 2 O (60 min after withdrawal of isoflurane, n =3 mice; Supplementary Fig. 7h–k ). In line with previous data, clusters of CaTs were completely suppressed by isoflurane ( Supplementary Fig. 7h–k , see also refs 42 , 43 ) and, in addition, entirely action potential-dependent ( Supplementary Fig. 7l–o ). GABAergic control of cortical network activity at P3–4 Using wide-field GCaMP3-based Ca 2+ imaging, we first examined whether cluster activity required intact NKCC1 and found that bath-applied bumetanide (50 μM) did not affect either cluster frequency ( f cluster ; P >0.2, n =5 mice, paired t -test; Fig. 5c and Supplementary Fig. 8a ) or cluster size (quantified as the mean number of active ROIs per cluster; P >0.9, paired t -test; Fig. 5d ). In addition, the frequency of spontaneous CaTs per ROI ( f ROI ) remained unaffected ( P >0.15, paired t -test; Fig. 5a,b ). Note that the same concentration of bumetanide (50 μM) strongly reduced the amplitude of CaTs evoked by exogenous GABA ( Fig. 2m–p ), confirming that bumetanide is able to penetrate to the ROI. Thus, our data suggest that GABA released synaptically during ongoing network activity does not contribute an essential excitatory drive to cluster activity. We next examined the effects of a use-dependent enhancement of intracortical GABA A R-mediated transmission. Bath application of the benzodiazepine diazepam (70 μM) strongly inhibited spontaneous network activity as reflected in a reduced f ROI ( P <0.001, n =6 mice, paired t -test; Fig. 5e,f ). This effect was mainly spatial in nature, since diazepam consistently reduced the mean cluster size ( P <0.01, paired t -test; Fig. 5h ), whereas f cluster was hardly affected ( P >0.1, paired t -test; Fig. 5g and Supplementary Fig. 8b ). We then investigated the contribution of endogenously released GABA by blocking GABA A Rs with gabazine (40 μM). This revealed a new type of synchronized and action potential-dependent activity ( Supplementary Fig. 7n,o ) frequently involving the entire field of view ( Fig. 5i ). Accordingly, f cluster was markedly elevated ( P <0.001, paired t -test; Fig. 5k and Supplementary Fig. 8c ) and cluster size strongly increased ( P <0.001, paired t -test; Fig. 5l ). As a result, gabazine induced a massive augmentation of f ROI ( P <0.001, paired t -test; Fig. 5i,j ). An inhibitory function of GABA A R activation by endogenous GABA in the upper CP was further supported by the observation that gabazine enhanced amplitudes of somatic CaTs induced by focal N-Methyl-D-aspartate (NMDA) application ( Supplementary Fig. 9 ). We finally asked whether extrasynaptic GABA A Rs [53] may contribute to the observed gabazine-induced disinhibition of cortical Ca 2+ cluster activity. We focussed on α5-subunit-containing GABA A Rs (α5-GABA A Rs) because of their early developmental expression [54] and the previously reported involvement in tonic GABAergic currents at the age investigated [55] . Using wide-field Ca 2+ imaging, we found that L-655,708 (1 μM), an α5-GABA A R-specific inverse agonist, disinhibited network activity as evidenced by an increase in f ROI ( P <0.05, n =5 mice, paired t -test; Fig. 5m,n ). This effect was largely spatial in origin because L-655,708 increased the mean cluster size ( P <0.01, paired t -test; Fig. 5p ) but did not significantly affect f cluster ( P >0.4, paired t -test; Fig. 5o and Supplementary Fig. 8d ). These data suggest that activation of α5-GABA A Rs contributes to the spatial confinement of cortical Ca 2+ clusters. In summary, we conclude that (at P3–4) GABAergic transmission has an inhibitory function at the network level. 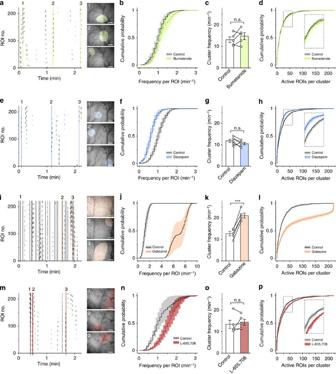Figure 5: GABAergic control of neocortical network activityin vivo. (a,e,i,m) Sample raster plots in the presence of bumetanide (a) diazepam (e) gabazine (i) and L-655,708 (m) from four different mice. Insets (right) show GCaMP3 fluorescence overlaid with binary area plots of Ca2+clusters as indicated on the left. Scale bars, 200 μm. (b,f,j,n) Distributions of the frequency of Ca2+transients per ROI. The mean (solid line)±s.e.m. (shaded area). (c,g,k,o) Cluster frequency (mean±s.e.m.) in control versus bumetanide (P>0.2,n=5 mice), control versus diazepam (P>0.1,n=6 mice), control versus gabazine (P<0.001,n=5 mice) and control versus L-655,708 (P>0.4,n=5 mice; pairedt-tests). Each pair of symbols represents a single animal. ***P<0.001, n.s., not significant. (d,h,l,p) Distributions of the number of active ROIs per Ca2+cluster event. Data presented as the mean (solid line)±s.e.m. (shaded area). Insets ind,h,pshow boxed region at higher magnification. Figure 5: GABAergic control of neocortical network activity in vivo . ( a , e , i , m ) Sample raster plots in the presence of bumetanide ( a ) diazepam ( e ) gabazine ( i ) and L-655,708 ( m ) from four different mice. Insets (right) show GCaMP3 fluorescence overlaid with binary area plots of Ca 2+ clusters as indicated on the left. Scale bars, 200 μm. ( b , f , j , n ) Distributions of the frequency of Ca 2+ transients per ROI. The mean (solid line)±s.e.m. (shaded area). ( c , g , k , o ) Cluster frequency (mean±s.e.m.) in control versus bumetanide ( P >0.2, n =5 mice), control versus diazepam ( P >0.1, n =6 mice), control versus gabazine ( P <0.001, n =5 mice) and control versus L-655,708 ( P >0.4, n =5 mice; paired t -tests). Each pair of symbols represents a single animal. *** P <0.001, n.s., not significant. ( d , h , l , p ) Distributions of the number of active ROIs per Ca 2+ cluster event. Data presented as the mean (solid line)±s.e.m. (shaded area). Insets in d , h , p show boxed region at higher magnification. Full size image Two independent lines of optical and electrophysiological evidence suggest that GABA acts as a depolarizing neurotransmitter in the developing (P3–4) mouse occipital neocortex. (1) In cell-attached current-clamp recordings, GABA was found to induce depolarization in most neurons examined. (2) When VGCC activation was pharmacologically enhanced using BayK 8644, GABA A R activation induced somatic CaTs in the majority of CP cells. Ad (1) Additional experiments in juvenile mice at P25–27 showed that GABA failed to depolarize the majority of more mature layer 2/3 neurons, thereby supporting the concept of a shift in GABA action during brain maturation [4] . At the same age, GABA A R-mediated hyperpolarization was detected in only one out of 10 neurons examined (in the presence of a membrane-permeable carbonic anhydrase inhibitor). The latter observation strongly suggests that shunting inhibition, rather than hyperpolarization, is the main form of inhibition in the juvenile/adult cortex in vivo (in agreement with previous in vitro data [12] , [21] ). Ad (2) Pharmacological inhibition of NKCC1 strongly reduced the amplitudes of GABA-evoked CaTs, implying an important role for secondary active chloride accumulation in GABAergic transmission in vivo . The latter observation indirectly supports the notion that GABA A R-dependent depolarization primarily results from a depolarizing chloride (rather than bicarbonate [56] ) flux. It should be noted here that drug superfusion of the exposed dura mater (referred to as bath application in the present study) circumvents the blood–brain barrier. This aspect might be particularly relevant for the NKCC1 blocker bumetanide that poorly penetrates the blood–brain barrier [57] . In line with the view that NKCC1-dependent chloride accumulation is functional in the intact brain, focal injection of bumetanide was recently reported to reduce the migration velocity of GABAergic interneurons in layer I at P0–3 in vivo [58] . In the presence of BayK 8644, we found that 55% and 95% of cells generated somatic CaTs in response to GABA and muscimol, respectively. Since GABA B Rs do not mediate hyperpolarizing postsynaptic responses in rodent neocortex until the end of the first postnatal week [59] , activation of metabotropic GABA receptors is inapplicable in explaining the difference. Potentially reflecting a differential degree of GABA A R activation (possibly related to the fact that GABA, but not muscimol, represents a substrate for GABA transporters), these data support the conclusion that GABAergic transmission is depolarizing in the majority of immature CP neurons at P3–4. In contrast, a previous study in cerebellar interneurons revealed that GABA A R activation could lead to a rise in [Ca 2+ ] i via an alternative mechanism involving a regulatory volume decrease reaction [60] . Because GABA A R-dependent CaTs in the present study were completely sensitive to the VGCC antagonist CdCl 2 , this scenario seems unlikely. Theoretically, a transient GABA A R-dependent hyperpolarization might activate an excitatory conductance (for example, hyperpolarization-activated I h or low-voltage-activated Ca 2+ channels) that, in turn, could induce a depolarization-dependent rise in [Ca 2+ ] i (ref. 61 ). The latter possibility could be largely ruled out by using cell-attached current-clamp recordings that revealed a monophasic time course of GABA-mediated depolarization in most cells examined. Under control conditions (that is, in the absence of BayK 8644), both epidural and local (that is, intraparenchymal) puff application of GABA A R agonists mostly failed to induce a distinct rise in [Ca 2+ ] i at P3–4. This finding is in striking contrast to previously reported in vitro data from the CP [5] , [13] , [30] , [41] , which we corroborated in the present study. The observation cannot be sufficiently explained by desensitization of GABA A Rs and/or VGCCs as a result of slow application kinetics since, in vitro , even bath application of GABA (leading to considerably slower [GABA] transients) reliably induced somatic CaTs at the same age [5] , [7] . In addition, synaptic stimulation in the presence of ionotropic glutamate receptor antagonists did not induce somatic CaTs as well. In agreement with the observed lack of GABA-induced CaTs, both puff application of GABA and afferent GABAergic synaptic stimulation failed to induce action potential firing. These data suggest that GABA A R-mediated depolarization in vivo is mostly subthreshold at P3–4, that is, lacks direct ( sensu stricto ) excitatory effects. Interestingly, the pharmacological properties of GABA-evoked CaTs in the presence of BayK 8644 were virtually identical to those previously reported from brain slice preparations [5] , [30] . This supports the notion that differential effects of GABA on [Ca 2+ ] i in vivo versus in vitro are (in terms of the underlying depolarization) likely quantitative, rather than qualitative, in nature. At present, it is unclear which factors underlie this discrepancy. Certainly, slow active chloride uptake in immature neurons [62] in conjunction with a higher chloride conductance in vivo versus in vitro , for example, due to synaptic [50] or extrasynaptic GABA A R activation, represents a potential candidate [25] . Whether traumatic injury might affect results obtained from in vitro preparations is currently highly debated [28] , [44] . What could be the developmental function of subthreshold-depolarizing GABAergic transmission in the immature cortex? Theoretical considerations and experimental evidence suggest, for instance, that the reversal potential for GABA A R-mediated currents (which itself is activity-dependent [24] ) contributes to the control of spike timing [63] . By modulating spike timing-dependent forms of synaptic plasticity, GABA-mediated depolarization might have developmental effects independent of a gross change in overall activity levels. Interestingly, a recent study proposed that depolarizing GABAergic transmission during early development controls critical-period plasticity in rat visual cortex [64] . Collectively, our data reveal that GABA A R activation triggers membrane depolarization in the majority of upper CP neurons at P3–4 in vivo . It should be stressed that GABA-mediated depolarization might even be more pronounced at earlier postnatal stages. In line with this idea, we found that at P1 GABA A R activation induced somatic CaTs in ∼ 9% of CP cells in the absence of BayK 8644. Hence, these data could potentially point to an excitatory action of GABA in a subset of neurons at this age. Clearly, further research is required to clarify whether or not this is the case. Previous electrophysiological and imaging studies identified retinal wave-triggered spindle bursts [50] or Ca 2+ waves [43] as the dominant network activity pattern in the intact rodent visual cortex. Using simultaneous wide-field Ca 2+ imaging and extracellular recording techniques, we show here that network Ca 2+ clusters and spindle bursts/delta waves represent homologous events. In line with previous studies from the rat visual cortex [50] , [51] , distinct gamma oscillations were not evident in the present study (as opposed to, for example, somatosensory and motor cortex [65] ). Our data further revealed that the generation of Ca 2+ clusters in the occipital cortex is essentially independent of NKCC1—in spite of its cellular effects (see above). Computational modelling and experimental studies in vitro have extensively characterized the conditions under which a subthreshold-depolarizing GABAergic conductance may facilitate action potential discharge (excitatory sensu lato ) or, alternatively, inhibit neuronal output [20] , [21] , [22] , [23] , [24] . Although not excluding excitatory sensu lato actions of GABA, our data are compatible with the view that these, if present, are not required to drive spontaneous cortical network activity. Moreover, our data are in agreement with a previous pharmacological characterization of spindle bursts in the somatosensory cortex [37] and suggest that the observed Ca 2+ clusters are not the in vivo counterpart of NKCC1-dependent giant depolarizing potentials in vitro , which do depend on depolarizing GABA actions as a promoter of glutamatergic transmission [11] , [12] . It therefore might be speculated that Ca 2+ clusters reported in the present study represent the in vivo analogue of so-called cortical early network oscillations recorded in vitro during the first postnatal week [11] , [13] from which, however, Ca 2+ clusters appear to differ in spatial extent. Focussing on P3–4, our data obviously do not exclude the possibility that NKCC1 (or even GABAergic depolarization) has a more accentuated role for the generation of in vivo activity patterns during earlier/later developmental periods and/or in other brain regions [36] . Furthermore, we could show that endogenous GABA acting via GABA A Rs exerts a powerful inhibition on cortical Ca 2+ clusters by constraining both their frequency of occurrence and their spatial extent. The latter is partially mediated by α5-GABA A Rs, pointing to a role of peri-/extrasynaptic GABAergic transmission [53] . Whether α5-GABA A Rs are activated in a phasic (by GABA spillover following synaptic release during Ca 2+ cluster activity) and/or tonic (by ambient GABA) manner remains an interesting open question. Our present findings contrast with several (but not all [11] ) in vitro studies showing that GABA A R blockade in cortical slices partially suppressed large-scale Ca 2+ waves [13] , [14] , [15] , but agrees well with previous data on spindle bursts in the intact somatosensory cortex [37] . Disinhibition due to the GABA A R blockade was also observed for focally evoked NMDA receptor-mediated responses in the upper CP. Combining measurements at the single-cell and network level, our data thereby show that, in vivo , depolarizing GABAergic transmission has additional inhibitory functions at the network level, likely via the GABA A R-dependent increase in membrane conductance (that is, shunting inhibition). This is in line with both conclusions derived from mathematical modelling and experimental in vitro data [22] , [23] . It has been hypothesized that, in the neonatal rodent visual cortex, the sequential activation of corresponding retinal and cortical domains is crucial for the proper establishment of retinotopic maps, as previously shown for the optic tectum [66] . Our data support the view that cortical GABAergic transmission is central in maintaining the spatiotemporal specificity of this co-activation. In summary, by extending previous in vitro investigations, our data identify GABA as a predominantly depolarizing (at the cellular level) and, at the same time, inhibitory (at the network level) neurotransmitter during early (P3–4) cortical development in vivo . Animals All animal procedures were performed with approval from the local government (registration number: 02-053/11, Thüringer Landesamt für Verbraucherschutz) and complied with international and European Union norms. Experiments were performed on C57BL/6J (two-photon Ca 2+ imaging and electrophysiological experiments) and Emx1 IREScre :GCaMP3 LSL (wide-field epifluorescence and two-photon imaging) mice at P3–4 ( n =92 mice), except for separate subsets of experiments at P1 ( n =3 mice) and P25–27 ( n =8 mice). Emx1 IREScre :GCaMP3 LSL mice were obtained by crossing homozygous female Emx1 IREScre mice [48] (The Jackson Laboratory, stock no. 005628) with homozygous male GCaMP3 LSL mice [49] (Ai38, The Jackson Laboratory, stock no. 014538). Surgical preparation For in vivo recordings, animals were deeply anaesthetized with isoflurane (3.5% for induction, 1–2% for maintenance) in pure oxygen and the skin overlying the skull locally infiltrated with 2% lidocaine (s.c.). Scalp and periosteum were removed, and a plastic chamber with a central hole (Ø 2–3 mm) was fixed on the skull using cyanoacrylate glue [67] , [68] . The recording chamber was tightly connected to the microscope stage and subsequently perfused with ACSF containing (in mM): 125 NaCl, 4 KCl, 25 NaHCO 3 , 1.25 NaH 2 PO 4 , 2 CaCl 2 , 1 MgCl 2 and 10 glucose (pH=7.4 at 35–36 °C; ACSF flow rate ∼ 3 ml min –1 ). A craniotomy ( ∼ 0.3–0.7 mm 2 for single-cell recordings, ∼ 1.0–1.4 mm 2 for wide-field imaging) was performed above the left occipital cortex using a 27G needle, except for recordings presented in Supplementary Fig. 7e–h . Care was taken not to damage the underlying dura mater. Anaesthesia and animal monitoring during recordings During in vivo recordings, body temperature was continuously monitored and maintained at close to physiological values (34–37 °C) by means of a heating pad. Spontaneous respiration was monitored using a differential pressure amplifier (Spirometer Pod and PowerLab 4/35, ADInstruments). For wide-field epifluorescence imaging, isoflurane was discontinued after completion of the surgical preparation and gradually substituted with the analgesic-sedative nitrous oxide (up to the fixed final N 2 O/O 2 ratio of 3:1). Experiments started ≥90 min after withdrawal of isoflurane. For two-photon Ca 2+ imaging, animals were either sedated with N 2 O (as above) or, to reduce the frequency of pup movements, anaesthetized with isoflurane (with or without N 2 O). Depth of anaesthesia was controlled by adjusting the dose of isoflurane (typically 0.5–1.2%) and/or the N 2 O/O 2 ratio (up to 3:1) to maintain a mean respiration rate of ∼ 90–110 min –1 . The latter anaesthetic regime was also used for single-cell electrophysiological recordings. For P3–4 mice, body weight before surgery was 2.31±0.07 g ( n =60), and weight loss during in vivo experiments (≤10 h) amounted to 1.45±0.14% ( n =50). Two-photon microscopy Multicell bolus loading [69] of cells with the AM-ester of the Ca 2+ indicator Oregon Green 488 BAPTA-1 (OGB1, 310–500 μM) was performed by pressure ejection (for 1–2 min at 40–50 kPa) using a patch pipette (3–7 MΩ, ∼ 150–300 μm below pia). To allow for de-esterification, recordings were performed at >1 h post-OGB1 AM injection. Imaging was performed using a Movable Objective Microscope (Sutter Instrument) controlled by the software MPScope 2.0 and custom-made software written in LabView (National Instruments). Fluorescence excitation at 800–830 nm (OGB1) or 920 nm (GCaMP3) was provided by a tunable Ti:Sapphire laser (Chameleon Ultra II, Coherent) using a × 20/1.0 NA water immersion objective (Olympus). Emission light was separated from excitation light using a 670-nm dichroic mirror (670 DCXXR, Chroma Technology), filtered at 535/50 nm and detected by a photomultiplier tube (H10770PA-40, Hamamatsu). Images were typically acquired at a frame rate of 11.6 Hz (256 × 256 pixels) or 3.4 Hz (512 × 512 pixels). Recordings were performed in the upper CP (usually <150 μm below pia). For analysis, fluorescence signals from cell somata (manually outlined in an average image of the pre-stimulus period) were, if possible, corrected for background fluorescence (calculated from the lumen of a cross-sectioned blood vessel) and expressed as relative changes from pre-stimulus levels (Δ F / F 0 ). Normalized rise slopes for glutamate-induced responses were calculated as follows: first, a two-term Boltzmann function was fitted to the Δ F / F 0 time series. Second, the maximum slope during the rising phase of the responses was determined from the fit and, finally, normalized to the amplitude of the response. Electrophysiological recordings Electrophysiological signals were acquired using an Axopatch 200B (patch-clamp) or Multiclamp 700B (patch-clamp and extracellular recordings) amplifier, a 16-bit AD/DA board (Digidata 1440A) and pClamp 10.2 (Molecular Devices). Signals were either low-pass-filtered at 2 kHz and sampled at 20 kHz in patch-clamp studies or band-pass-filtered at 0.1–6,000 Hz and sampled at 100 kHz in extracellular recordings. A shadow-patching approach was used to visually target recordings to the upper CP. To this end, pipette solutions were supplemented with Alexa Fluor 488 (100 or 500 μM) and visualized by two-photon excitation at 920–930 nm. All cells included in the analysis were identified as neurons on the basis of (I) their ability to generate action potentials/currents (in whole-cell/cell-attached mode) either spontaneously or evoked (by voltage jumps or puff-applied glutamate) or (II) in some cases (at P25–27) by the presence of postsynaptic currents in the whole-cell mode. To evaluate the polarity of GABA-induced membrane potential changes, tight-seal cell-attached current-clamp recordings were performed ( I =0 mode of the amplifier) [30] , [40] , [70] . Recording pipettes (3–7 MΩ) were filled with one of the following solutions (in mM): (1) 140 K + gluconate, 10 HEPES, 11 EGTA, 1 CaCl 2 and 2 MgCl 2 (pH 7.25) or (2) 135 K + gluconate, 5 KCl, 10 HEPES, 11 EGTA, 1 CaCl 2 and 2 MgCl 2 (pH 7.25). Total resistance measured in the cell-attached mode was 6.5±0.31 GΩ ( n =15) at P3–4 and 6.3±0.46 GΩ ( n =16) at P25–27. To quantify agonist-induced changes in membrane resistance, whole-cell voltage-clamp recordings were performed at a holding potential of –70 mV (not corrected for liquid junction potentials; pipette solutions as above). Series resistance ( R s ) was estimated from the peak current in response to hyperpolarizing (–10 mV, 50 ms) voltage steps, and membrane resistance ( R m ) from the respective steady-state current ( I ss ) assuming that R m and R s additively contribute to I ss . In this set of experiments, R s amounted to 42±1.9 MΩ, reflecting an R s / R m ratio of 6.8±1.0% ( n =9). For measurements of agonist-induced action currents, loose-patch (seal resistance <100 MΩ) or tight-seal (>1 GΩ) cell-attached recordings were performed in the voltage-clamp mode using glass pipettes filled with the following solution (in mM): 150 NaCl, 4 KCl and 10 HEPES (pH 7.4). Holding current was manually zeroed before each experiment. Extracellular recordings were performed using glass pipettes beveled to a resistance of 200–500 kΩ. Recording pipettes were positioned in the upper CP under two-photon guidance. For synchronization with wide-field Ca 2+ imaging, a light-emitting diode was used to deliver 2-ms light pulses at intervals of 1 min. Electrical stimulation For electrical stimulation of afferent fibres, a low-resistance (200–500 kΩ) glass electrode was positioned in the upper CP under two-photon guidance. Each trial of stimulation consisted of 25 pulses (40–100 V, 200 μs) delivered at 50 Hz using an isolated pulse stimulator (Model 2100, A-M Systems). In two-photon Ca 2+ imaging experiments, cells were classified as responsive if, within an interval of 2.15 s (25 frames) after the start of stimulation, Δ F / F 0 exceeded a threshold of three times the s.d. of the baseline noise for ≥3 frames (this was separately carried out for each single trial and the averaged Δ F/F 0 time series). For patch-clamp recordings, we first performed multicell bolus loading with OGB1 to identify the responsive region (in standard ACSF) within which cell-attached recordings were subsequently conducted. Synaptically evoked action currents were differentiated from antidromically induced responses on the basis of their latency (>2 ms). Wide-field epifluorescence microscopy One-photon excitation of the genetically encoded Ca 2+ indicator GCaMP3 was provided by a xenon arc lamp (Lambda LS, Sutter Instrument) coupled via a liquid light guide to the epifluorescence port of a Movable Objective Microscope (Sutter Instrument) and filtered at 472/30 nm. Emission was separated from excitation light at 495 nm and long-pass-filtered at 496 nm (AHF Analysentechnik). Images were acquired using a × 10/0.3 NA water immersion objective (Zeiss) and a 12- bit Rolera-XR camera (QImaging) operated by the software Streampix 5 (NorPix). Frame rate was set to 74.14 Hz using 4 × 4 hardware binning (170 × 130 pixels; field of view: 1,134 × 867 μm). Recording time per condition typically amounted to 18.0 min (range: 13.2–22.4 min). For analysis, periods of movement artefacts were first identified by visual inspection of raw image sequences and discarded since they frequently resulted in obviously false-positive detection results. Image sequences were then binned (10 × 10), giving rise to a regular grid of 17 × 13=221 ROIs (ROI dimensions: 66.7 × 66.7 μm). Next, intensity-versus-time plots were extracted using ImageJ 1.47 ( http://rsbweb.nih.gov/ij/ ). Unbiased peak detection of spontaneous CaTs was performed using a template-matching algorithm implemented in pClamp 10.2. ‘Clusters’ of CaT peaks were defined on a temporal basis as follows. Extracted peak times were binned (bin width=5 frames, ∼ 67.4 ms) and neighbouring non-empty bins (that is, bins with ≥1 peak) were considered to belong to a common temporal cluster if they were separated by less than two empty bins. The mean frequencies of CaTs per ROI as well as the mean cluster frequencies were calculated as the ratio of number of events per corrected recording time (that is, total recording time minus cumulative movement artefact-associated recording time). Drug application In vivo epidural puff application of agonists (100 mM glutamate, 100 mM GABA, 5 mM muscimol and 5 mM baclofen) or ACSF at a nominal pressure of 69 kPa (Toohey Spritzer) was performed via a patch pipette (typically 3–6 MΩ) positioned in close proximity to the intact dura. Substances for application were dissolved in extracellular solution of the respective control condition. In electrophysiological experiments, a ‘standard’ GABA or glutamate puff of constant duration (5 s) was used. In these experiments, the application pipette additionally included the red fluorescent dye Alexa Fluor 594 (100 μM; excited at 830 nm). Trials were accepted for analysis if application was associated with a distinct increase in fluorescence in the immediate vicinity of the recorded neuron, but otherwise discarded. In two-photon Ca 2+ imaging experiments involving epidural applications, fluorescent dyes were omitted from application solutions. Instead, the following procedure was applied: (I) epidural puff application of glutamate leads to spatially confined cell activation because of limited agonist diffusion distance. Therefore, we used puff application of glutamate to validate proper pipette positioning. Within the activation volume, almost all cells (>95%) did respond to glutamate. (II) The duration of the glutamate puff was adjusted such that the mean Δ F / F 0 was in the order of 1.0–1.5. This duration was defined as t short (for experiments in Fig. 2b–d , t short ranged from 0.3 to 2.0 s). Setting the application time to 67% of t short reduced the amplitude of full-field responses to 59.0±3.4% ( n =4 mice). (III) The glutamate-containing pipette was replaced by a second pipette that contained a GABA receptor agonist, and the experiment was repeated (again using t short ). For experiments depicted in Fig. 2e–p, a prolonged GABA application time was used according to the definition: t long =5 × t short . An analogous procedure was applied during in vitro Ca 2+ imaging experiments ( Supplementary Fig. 3 ). To reduce differences in effective concentrations, agonist concentrations were reduced (1 mM glutamate, 1 mM GABA) so as to compensate for the lack of diffusional barriers in the slice preparation that are present in vivo (for example, dura mater). Moreover, application times ( t short ) were adjusted such that amplitudes of glutamate-induced CaTs in vitro were similar to those measured in vivo . For in vivo experiments involving local pressure application of GABA (10 mM) or glutamate (10 mM), pipettes (typically 10–15 MΩ) were supplemented with Alexa Fluor 594 (20 μM) to verify solution outflow. Local puff application (30 or 40 ms) resulted in a circumscribed mechanical artefact close to the pipette tip (area=1.2±0.1 × 10 3 μm 2 , n =18 trials). Cells located within this area were excluded from further analysis. A cell was considered responsive to glutamate ( in vivo and in vitro) if glutamate-induced Δ F / F 0 ≥0.2. Under control conditions, responsiveness to GABA was defined on the basis of a threshold criterion derived as follows: the mean standard deviation of the baseline noise (s.d.) was 0.05 for both t short and t long at P1. At P3–4, s.d. amounted to 0.06 for t short and 0.07 for t long . Cells were classified as responsive to GABA if (I) Δ F / F 0 >0.08 (set constant for all cells analysed) and, to minimize the number of false positives, (II) Δ F / F 0 >3 × s.d. (here s.d. refers to the specific cell analysed). Preparation of acute brain slices Animals were decapitated under deep isoflurane anaesthesia. The brain was removed quickly and transferred into ice-cold saline containing (in mM): 125 NaCl, 4 KCl, 10 glucose, 1.25 NaH 2 PO 4 , 25 NaHCO 3 , 0.5 CaCl 2 and 2.5 MgCl 2 , bubbled with 5% CO 2 /95% O 2 (pH 7.4). Coronal slices (350 μm) comprising the occipital cortex were cut on a vibratome (VT1200 S, Leica) and stored for at least 1 h before use at room temperature in ACSF. For recordings, slices were placed into a submerged-type recording chamber (ACSF flow rate ∼ 3 ml min –1 ) on the stage of a Movable Objective Microscope (see above). All experiments were performed at 35–36 o C. Chemicals Chemicals were obtained from Sigma (GABA, glutamate sodium salt, muscimol, APV, bumetanide, cadmium chloride, 6,7-dinitroquinoxaline-2,3(1H,4H)-dione (DNQX), EZA, L-655,708, NMDA, picrotoxin, gabazine), Tocris [( R )-baclofen, ( S )-(-)-BayK 8644] and Biotrend (TTX). Diazepam was obtained from Krewel Meuselbach (Valocordin) and Caesar & Loretz. Statistics Statistical analyses were performed using OriginPro 8/9, Microsoft Excel 2003/2010 and SPSS Statistics 19. All data are reported as mean±s.e.m. Unless otherwise stated, the statistical parameter n refers to the number of animals in Ca 2+ imaging experiments or to the number of cells in electrophysiological recordings. The Shapiro–Wilk test was used to test for the normality of data. Parametric testing procedures were applied for normally distributed data; otherwise nonparametric tests were used. P values (two-tailed tests) <0.05 were considered statistically significant. How to cite this article: Kirmse, K. et al . GABA depolarizes immature neurons and inhibits network activity in the neonatal neocortex in vivo . Nat. Commun. 6:7750 doi: 10.1038/ncomms8750 (2015).